Haemodynamic and extracellular matrix cues regulate the mechanical phenotype and stiffness of aortic endothelial cells Endothelial cells (ECs) lining blood vessels express many mechanosensors, including platelet endothelial cell adhesion molecule-1 (PECAM-1), that convert mechanical force into biochemical signals. While it is accepted that mechanical stresses and the mechanical properties of ECs regulate vessel health, the relationship between force and biological response remains elusive. Here we show that ECs integrate mechanical forces and extracellular matrix (ECM) cues to modulate their own mechanical properties. We demonstrate that the ECM influences EC response to tension on PECAM-1. ECs adherent on collagen display divergent stiffening and focal adhesion growth compared with ECs on fibronectin. This is because of protein kinase A (PKA)-dependent serine phosphorylation and inactivation of RhoA. PKA signalling regulates focal adhesion dynamics and EC compliance in response to shear stress in vitro and in vivo . Our study identifies an ECM-specific, mechanosensitive signalling pathway that regulates EC compliance and may serve as an atheroprotective mechanism that maintains blood vessel integrity in vivo . Mechanical forces influence nearly all aspects of cell behaviour, including apoptosis, transcription and translation, differentiation and cell migration [1] , [2] , [3] , [4] , [5] . The mechanical environment of a cell consists of both cell-generated (endogenous) and applied (exogenous) forces. Endogenous forces are generated when a cell pulls on the extracellular matrix (ECM) or its neighbours via its cytoskeleton. Examples of exogenous forces include the mechanical force of shear stress applied on endothelial cells (ECs) due to blood flow, as well as the stretching of vascular cells due to blood pressure. It is now well accepted that mechanical stresses determine the mechanical properties of cells, which, in turn, influence cell function in both physiology and disease. Nevertheless, the relationship between force and biological response remains elusive. Various methods have been used to apply exogenous forces to cells [6] , [7] , [8] . These studies have revealed that when force is applied to mechanosensitive proteins, cells respond by increasing their stiffness. This is a physiological response that is required in order to resist the applied force; however, increased stiffness is also associated with pathologies such as cardiovascular disease and cancer [9] , [10] , [11] . We and others have demonstrated that the stiffening response requires the coordination of numerous signalling cascades, including activation of the small GTPase RhoA [6] , [7] , [12] . Effectors downstream of the GTPase coordinate changes in the actin cytoskeleton and focal adhesions in an effort resist the applied force [12] . While much work has focused on integrin-mediated force transduction, recent work has highlighted other mechanosensitive proteins, such as cadherins and platelet endothelial cell adhesion molecule-1 (PECAM-1 (refs 5 , 12 , 13 , 14 )). PECAM-1 functions as a mechanosensor in the endothelium and activates a number of intracellular signalling cascades in response to the haemodynamic force of shear stress [15] . We recently reported that ECs adherent on fibronectin (FN) generate an adaptive stiffening response when tension is applied to PECAM-1 (ref. 12 ), and this response is dependent on integrin ligation with the underlying ECM. Integrin heterodimers differ in their ECM specificity based on their α/β subunit composition and therefore bind to distinct ECM proteins. Several studies have reported matrix-specific signalling through different integrin subtypes within the endothelium [16] , [17] , [18] . Throughout most of the vasculature, collagen (CL) and laminins are the predominant ECM proteins. However, distinct regions of the vasculature are rich in FN deposition and therefore differ in matrix composition. Variances in matrix composition along blood vessels permit the activation of ECM-specific signalling cascades in localized regions of the vasculature. For instance, fluid shear stress activates protein kinase A (PKA) in ECs adherent on CL, whereas PKA activity is unaffected when ECs adherent on FN are exposed to shear stress [18] . While ECM-specific signalling cascades have been identified, how these divergent signalling pathways affect mechanical signalling, cell mechanics and cellular functions are not understood. Here we investigate how the ECM identity and signalling through discrete integrin subtypes influences the cellular response to tension on PECAM-1. We reveal that the ECM composition has a profound effect on EC stiffness, both in vitro and in vivo in the haemodynamic environment of the vessel. We identify that CL-dependent and Gα s -mediated activation of PKA in response to mechanical force on PECAM-1 negatively regulates RhoA activity. Furthermore, we show that PKA-mediated inhibition of RhoA modulates the EC force response and focal adhesion dynamics in vitro and in vivo to, ultimately, dampen EC stiffness in the CL-rich descending aorta. The ECM determines the mechanoresponse to force on PECAM-1 In order to investigate the role of ECM composition on the mechanical response to tension on PECAM-1, we utilized magnetic tweezers to apply pulsatile force to ECs adherent on FN or CL. ECs incubated with anti-PECAM-1-coated paramagnetic beads were subjected to 2-s pulses of force over a 2-min time course ( Fig. 1a ). In ECs adherent on FN, application of successive pulses of force on PECAM-1 resulted in a significant decrease in bead displacement during latter pulses ( Fig. 1b ). This observed reduction in bead displacement is indicative of adaptive stiffening and consistent with previous work [12] . Surprisingly, when ECs adherent on CL were stimulated with the identical force regimen, we could not detect a significant change in pulse-to-pulse bead displacement, suggesting that the cells do not generate a force response in this context ( Fig. 1b ). Absolute displacement of anti-PECAM-1-coated beads during the first pulse of force was nearly identical on both FN and CL ( Supplementary Fig. 1 ). These results indicate that ECs adherent on FN or CL differ dramatically in their ability to respond to exogenous force application. Work from our group and others has demonstrated that the adaptive cellular stiffening response is mediated, in part, by an increase in focal adhesions that function to resist the applied force [12] , [19] . We assessed the focal adhesion profile in ECs plated on FN and CL before and after force manipulation. As previously reported, ECs adherent on FN exhibited robust focal adhesion growth in response to force on PECAM-1 ( Fig. 1c ). Conversely, and in agreement with the magnetic tweezers data, focal adhesion size or number did not significantly increase in ECs adherent on CL following force application. Taken together, these data indicate that the ECM composition has a profound effect on the cellular response to tension on PECAM-1. ECs adherent on FN generate an adaptive stiffening response, accompanied by significant focal adhesion growth, whereas ECs adherent on CL do not generate a significant force response or restructure focal adhesions in response to tension on PECAM-1. 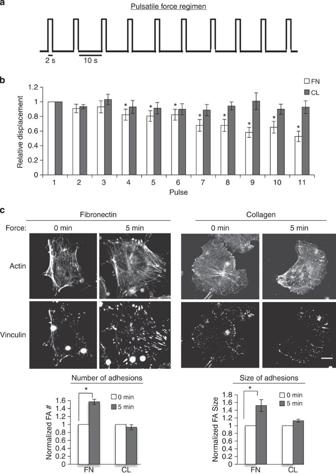Figure 1: ECM composition determines the cellular response to tension on PECAM-1. (a) Pulsatile force regimen applied with magnetic tweezers, consisting of a 2-s, 100-pN pulse of force, followed by a 10-s period of rest, repeated over a 2-min time course. (b) Average relative anti-PECAM-1-coated bead displacements induced by pulsatile force regimen. ECs were seeded on FN or CL 4 h before incubation with magnetic beads. Average displacements were calculated relative to the first pulse of force. (n>30 beads per condition from three independent experiments). Error bars represent s.e.m., *P<0.05 using a Student’st-test. (c) Adherent ECs on FN or CL were incubated with anti-PECAM-1-coated magnetic beads and subjected to force with a permanent magnet for the indicated times. ECs were fixed-stained with phalloidin and an anti-vinculin antibody to mark focal adhesions. Focal adhesion number and size were quantified using the NIH ImageJ software. Values were normalized to the FN ‘No Force’ condition.n>30 cells per condition from three independent experiments, *P<0.05 using a Student’st-test, scale bar=10 μm. Figure 1: ECM composition determines the cellular response to tension on PECAM-1. ( a ) Pulsatile force regimen applied with magnetic tweezers, consisting of a 2-s, 100-pN pulse of force, followed by a 10-s period of rest, repeated over a 2-min time course. ( b ) Average relative anti-PECAM-1-coated bead displacements induced by pulsatile force regimen. ECs were seeded on FN or CL 4 h before incubation with magnetic beads. Average displacements were calculated relative to the first pulse of force. ( n >30 beads per condition from three independent experiments). Error bars represent s.e.m., * P <0.05 using a Student’s t -test. ( c ) Adherent ECs on FN or CL were incubated with anti-PECAM-1-coated magnetic beads and subjected to force with a permanent magnet for the indicated times. ECs were fixed-stained with phalloidin and an anti-vinculin antibody to mark focal adhesions. Focal adhesion number and size were quantified using the NIH ImageJ software. Values were normalized to the FN ‘No Force’ condition. n >30 cells per condition from three independent experiments, * P <0.05 using a Student’s t -test, scale bar=10 μm. Full size image Phosphoinositide 3-kinase (PI3K) is a critical regulator of PECAM-1-mediated adaptive stiffening on FN by allowing integrin activation and downstream activation of RhoA [12] . In order to examine PI3K activation in ECs adherent on CL, anti-PECAM-1-coated paramagnetic beads bound to ECs expressing a GFP-PH fusion protein (which serves as a sensor for PI3–lipids) were subjected to force using a permanent ceramic magnet. Brief force application induced rapid PI3K activation around anti-PECAM-1-coated beads ( Supplementary Fig. 2a ) at levels similar to those previously reported in ECs adherent on FN [12] . These results suggest that the impaired mechanical response on CL is not because of insufficient PI3K activation. In order to assess force-dependent changes in CL-binding integrin (α2β1) activity, ECs adherent on CL were subjected to force and immunostained with an antibody that recognizes ligated β1 integrins. ECs exhibited transient but robust integrin activation after force application ( Supplementary Fig. 2b ), suggesting that the lack of a mechanical response in ECs adherent on CL may be because of divergent signalling downstream of CL-binding integrins. The ECM regulates mechanosensitive PKA and RhoA activation Activation of the small GTPase RhoA is known to be important for the cellular stiffening response [6] , [7] , [12] . Importantly, RhoA activation in response to tension on PECAM-1 requires integrin activation and ligation with the underlying ECM [12] . Although cells on CL exhibited significant integrin activation in response to tensional force on PECAM-1, we wanted to evaluate whether downstream RhoA activation was affected by ECM composition. Tension on PECAM-1 resulted in robust, but transient, activation of RhoA, as levels of GTP-bound RhoA increased at 5 min of force but returned to basal levels by 30 min of force ( Fig. 2a ). This transient response is in striking contrast to the prolonged RhoA activation that occurs when tension is applied to ECs adherent on FN ( Fig. 2b ). 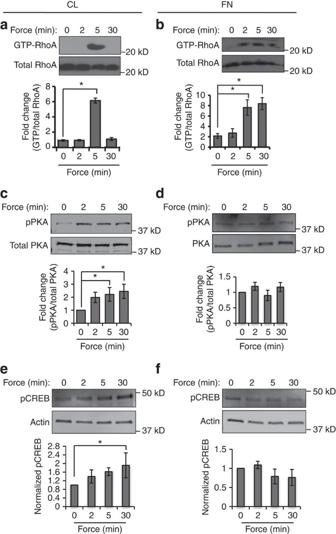Figure 2: ECM composition regulates mechanosensitive activation of the PKA-RhoA pathway. (a–f) Tension was applied to anti-PECAM-1-coated beads using a permanent ceramic magnet for the indicated times, and (a) active RhoA (RhoA-GTP) was isolated from EC adherent on CL with GST-RBD and analysed using western blot (n=5). (b) Active RhoA (RhoA-GTP) was isolated from EC adherent on FN with GST-RBD and analysed using western blot (n=5). (c) Cell lysates from ECs attached to CL were subjected to SDS–PAGE and immunoblotted for phospho (Tyr197) and total PKA (n=3). (d) Cell lysates from ECs adherent to FN were subjected to SDS–PAGE and immunoblotted for phospho (Tyr197) and total PKA (n=3). (e) Cell lysates from ECs adhered to CL were subjected to SDS–PAGE and immunoblotted for phospho-CREB (Ser133) and actin (n=3). (f) Cell lysates from ECs adherent on FN were subjected to SDS–PAGE and immunoblotted for phospho-CREB (Ser133) and actin (n=3). Bar graphs display averages from at least three independent experiments and error bars indicate s.e.m, *P<0.05 using a Student’st-test. Figure 2: ECM composition regulates mechanosensitive activation of the PKA-RhoA pathway. ( a – f ) Tension was applied to anti-PECAM-1-coated beads using a permanent ceramic magnet for the indicated times, and ( a ) active RhoA (RhoA-GTP) was isolated from EC adherent on CL with GST-RBD and analysed using western blot ( n =5). ( b ) Active RhoA (RhoA-GTP) was isolated from EC adherent on FN with GST-RBD and analysed using western blot ( n =5). ( c ) Cell lysates from ECs attached to CL were subjected to SDS–PAGE and immunoblotted for phospho (Tyr197) and total PKA ( n =3). ( d ) Cell lysates from ECs adherent to FN were subjected to SDS–PAGE and immunoblotted for phospho (Tyr197) and total PKA ( n =3). ( e ) Cell lysates from ECs adhered to CL were subjected to SDS–PAGE and immunoblotted for phospho-CREB (Ser133) and actin ( n =3). ( f ) Cell lysates from ECs adherent on FN were subjected to SDS–PAGE and immunoblotted for phospho-CREB (Ser133) and actin ( n =3). Bar graphs display averages from at least three independent experiments and error bars indicate s.e.m, * P <0.05 using a Student’s t -test. Full size image PKA has been implicated as a negative regulator of RhoA activity. The kinase can phosphorylate RhoA at serine 188 (ref. 20 ), and phosphorylation of this residue promotes association of the GTPase with guanine dissociation inhibitor. ECs exhibit mechanosensitive and matrix-specific activation of PKA, such that the kinase is activated in ECs adherent on CL in response to the mechanical stimulus of fluid shear stress but not activated in ECs adherent on FN [18] . Thus, we hypothesized that PKA may be differentially regulated in response to tension on PECAM-1, depending on the identity of the underlying ECM. In agreement with our hypothesis, when tension was applied to PECAM-1 on cells adherent to CL, we observed a significant force-dependent increase in PKA phosphorylation ( Fig. 2c ). However, we did not detect a significant change in PKA activity when cells on FN were subjected to force ( Fig. 2d ). In further support of matrix-specific activation of PKA, we also detected CL-specific activation of the downstream transcription factor cAMP-response element-binding protein (CREB), while CREB phosphorylation levels did not change in cells adherent on FN ( Fig. 2e,f ). PKA activation is mediated by Gα s -dependent signalling PKA exists as a holoenzyme that comprises two regulatory subunits bound to two catalytic subunits. Under low levels of cAMP, the regulatory subunits remain intact and holds the holoenzyme inactive. However, when the intracellular cAMP concentration increases, the nucleotide binds the regulatory subunits and releases the active catalytic subunits. We assessed whether mechanical tension on PECAM-1 results in increased cAMP levels and examined the role of the ECM in this activation. Consistent with our PKA data, we detected a significant force-dependent increase in cAMP levels in ECs adherent to CL, while levels remained unchanged in ECs attached to FN ( Fig. 3a ). These data suggest that matrix-specific differences in PKA activity are likely mediated by differential cAMP production. 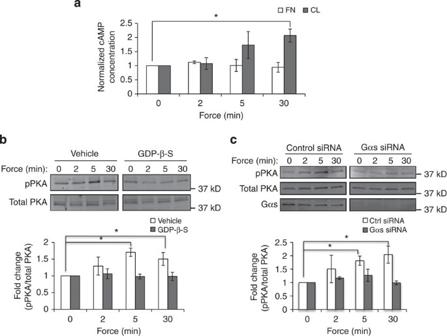Figure 3: CL-specific mechanosensitive PKA activation is mediated by Gαs-dependent cAMP production. (a–e) Tension was applied to anti-PECAM-1-coated beads using a permanent ceramic magnet for the indicated times, and (a) cAMP levels were measured by non-radioactive, competitive immunoassay (n=3). (b) ECs adherent on CL were pretreated with vehicle or GDP-β-S (20 μM, 30 min), subjected to force and processed for SDS–PAGE. Lysates were immunoblotted for phospho (Tyr197) PKA and total PKA (n=3). (c) ECs adherent on CL were transfected with control or Gαs-specific siRNAs. Ninety-six hours after transfection, ECs were subjected to force and processed for SDS–PAGE. Lysates were immunoblotted for phospho (Tyr197) PKA and total PKA (n=3). Bar graphs display averages from at least three independent experiments and error bars indicate s.e.m, *P<0.05 (Student’st-test). Figure 3: CL-specific mechanosensitive PKA activation is mediated by Gα s -dependent cAMP production. ( a – e ) Tension was applied to anti-PECAM-1-coated beads using a permanent ceramic magnet for the indicated times, and ( a ) cAMP levels were measured by non-radioactive, competitive immunoassay ( n =3). ( b ) ECs adherent on CL were pretreated with vehicle or GDP-β-S (20 μM, 30 min), subjected to force and processed for SDS–PAGE. Lysates were immunoblotted for phospho (Tyr197) PKA and total PKA ( n =3). ( c ) ECs adherent on CL were transfected with control or G α s -specific siRNAs. Ninety-six hours after transfection, ECs were subjected to force and processed for SDS–PAGE. Lysates were immunoblotted for phospho (Tyr197) PKA and total PKA ( n =3). Bar graphs display averages from at least three independent experiments and error bars indicate s.e.m, * P <0.05 (Student’s t -test). Full size image We next set out to investigate the mechanism of cAMP production on CL. cAMP production is often stimulated via Gα s -associated G-protein-coupled receptors that promote production of the nucleotide via activation of adenylyl cyclase. In order to test whether force-dependent PKA activation on CL was mediated by a G-protein-coupled receptor, ECs were pretreated with a general G-protein inhibitor (GDP-β-S) before force application on PECAM-1. Cells treated with vehicle displayed a significant increase in pPKA levels, while inhibition of G-protein signalling abolished force-dependent PKA activation on CL ( Fig. 3b ). Similarly, G-protein inhibition also blocked force-induced CREB phosphorylation in ECs attached to CL ( Supplementary Fig. 3 ). To specifically test for involvement of Gα s -dependent signalling, ECs were depleted of Gα s using specific short interfering RNAs (siRNAs). ECs adherent to CL and lacking Gα s did not display mechanosensitive activation of PKA, while control cells demonstrated an increase in pPKA levels in response to force on PECAM-1 ( Fig. 3c ). Therefore, our data suggest that CL-specific mechanosensitive activation of Gα s signalling results in matrix-specific cAMP production and subsequent activation of PKA. Mechanically induced PKA activity negatively regulates RhoA ECs attached to CL do not generate a mechanical response when tension is applied to PECAM-1 ( Fig. 1 ) and show differential activation of the PKA and RhoA pathways, when compared with cells adherent on FN ( Fig. 2 ). Given that PKA-dependent phosphorylation of RhoA has been shown to negatively regulate activity of the GTPase in other systems, we hypothesized that PKA phosphorylates RhoA and attenuates force-dependent RhoA activation in ECs adherent on CL. In order to test this hypothesis, levels of RhoA serine phosphorylation following force application on PECAM-1 were assessed with immunoprecipitation and immunoblot analyses ( Fig. 4a ). Indeed, ECs exhibited force-induced serine phosphorylation in response to tension on PECAM-1, suggesting that RhoA may be inactivated via serine phosphorylation at later time points. In order to test whether PKA mediates force-induced serine phosphorylation of RhoA, ECs were pretreated with the PKA inhibitor (PKI), before mechanical stimulation. Consistent with our hypothesis, PKA inhibition completely abolished force-dependent RhoA phosphorylation ( Fig. 4b ). These data indicate that force-induced activation of PKA promotes phosphorylation and inactivation of RhoA in ECs adherent on CL. Thus, we reasoned that abrogation of PKA signalling and, therefore, inhibition of RhoA serine phosphorylation should also influence levels of active or GTP-bound RhoA in response to tension on PECAM-1. In agreement with our hypothesis, blockade of PKA signalling resulted in robust and sustained activation of RhoA ( Fig. 4c ). Taken together, these data indicate that PKA activation modulates RhoA serine phosphorylation and, thus, activity of the GTPase in response to tension on PECAM-1. 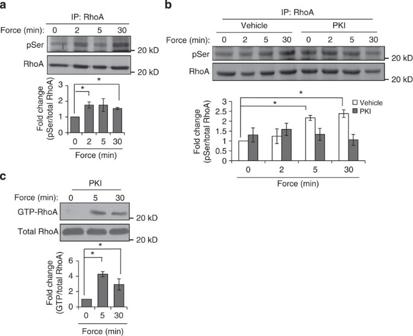Figure 4: Mechanically induced PKA activity negatively regulates RhoA. (a–c) Tension was applied to anti-PECAM-1-coated beads using a permanent ceramic magnet for the indicated times, and (a) total RhoA protein was immunoprecipitated from cell lysates and immune complexes were subjected to SDS–PAGE, followed by immunoblotting with phosphoserine and RhoA antibodies (n=3). (b,c) ECs were treated with PKI (20 μM for 1 h) or dimethylsulphoxide (DMSO), and tension was applied to anti-PECAM-1-coated beads using a permanent ceramic magnet for the indicated times. (b) Total RhoA protein was immunoprecipitated from cell lysates and immune complexes were subjected to SDS–PAGE, followed by immunoblotting with phosphoserine and RhoA antibodies (n=3). (c) Active RhoA (RhoA-GTP) was isolated with GST-RBD and analysed using western blot (n=3). Bar graphs display averages from at least three independent experiments and error bars indicate s.e.m, *P<0.05 using a Student’st-test. Figure 4: Mechanically induced PKA activity negatively regulates RhoA. ( a – c ) Tension was applied to anti-PECAM-1-coated beads using a permanent ceramic magnet for the indicated times, and ( a ) total RhoA protein was immunoprecipitated from cell lysates and immune complexes were subjected to SDS–PAGE, followed by immunoblotting with phosphoserine and RhoA antibodies ( n =3). ( b , c ) ECs were treated with PKI (20 μM for 1 h) or dimethylsulphoxide (DMSO), and tension was applied to anti-PECAM-1-coated beads using a permanent ceramic magnet for the indicated times. ( b ) Total RhoA protein was immunoprecipitated from cell lysates and immune complexes were subjected to SDS–PAGE, followed by immunoblotting with phosphoserine and RhoA antibodies ( n =3). ( c ) Active RhoA (RhoA-GTP) was isolated with GST-RBD and analysed using western blot ( n =3). Bar graphs display averages from at least three independent experiments and error bars indicate s.e.m, * P <0.05 using a Student’s t -test. Full size image PKA inhibition confers mechanoresponsiveness to ECs on CL In light of these data, we hypothesized that inhibition of PKA (and prolonged activation of RhoA) may confer the stiffening response to ECs adherent on CL. To address this, we pretreated ECs with PKI before stimulating PECAM-1 in the magnetic tweezers system. Control ECs did not respond to tension on PECAM-1 (similar to Fig. 1b ). In contrast, inhibition of PKA signalling resulted in a rapid and significant adaptive stiffening response ( Fig. 5a ). In addition, knockdown of the catalytic subunit of PKA using specific siRNAs also induced a significant stiffening response in ECs plated on CL ( Supplementary Fig. 4 ). These data suggest that prolonged activation of RhoA is sufficient to restore mechanical responsiveness to tension on PECAM-1. In order to examine whether inhibition of PKA permitted force-induced growth of focal adhesions in cells attached to CL, ECs pretreated with PKI were subjected to force and immunostained for the focal adhesion protein vinculin. In agreement with our magnetic tweezers studies, blockade of PKA signalling resulted in a significant increase in focal adhesion size and number, whereas vehicle-treated ECs did not exhibit significant focal adhesion growth ( Fig. 5b ). Thus, our data indicate that suppression of PKA signalling restores the mechanical response to tension on PECAM-1. 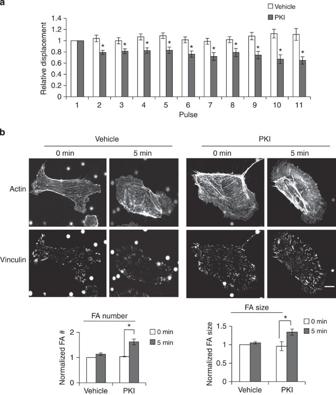Figure 5: Inhibition of PKA confers mechanical responsiveness to ECs on CL. (a,b) ECs were pretreated with PKI (20 μM) or vehicle for 1 h, and (a) pulsatile forces were applied to PECAM-1 with magnetic tweezers. Average relative anti-PECAM-1-coated bead displacements induced by pulsatile force regimen. Average displacements were calculated relative to the first pulse of force. (n>20 beads per condition from three independent experiments). (b) Anti-PECAM-1-coated magnetic beads were subjected to force with a permanent ceramic magnet for the indicated times. ECs were fixed-stained with phalloidin and an anti-vinculin antibody to mark focal adhesions. Focal adhesion number and size were quantified using the NIH ImageJ software. Values were normalized to the vehicle ‘No Force’ condition.n>30 cells per condition from three independent experiments, *P<0.05 using Student’st-test, scale bar=10 μm. Figure 5: Inhibition of PKA confers mechanical responsiveness to ECs on CL. ( a , b ) ECs were pretreated with PKI (20 μM) or vehicle for 1 h, and ( a ) pulsatile forces were applied to PECAM-1 with magnetic tweezers. Average relative anti-PECAM-1-coated bead displacements induced by pulsatile force regimen. Average displacements were calculated relative to the first pulse of force. ( n >20 beads per condition from three independent experiments). ( b ) Anti-PECAM-1-coated magnetic beads were subjected to force with a permanent ceramic magnet for the indicated times. ECs were fixed-stained with phalloidin and an anti-vinculin antibody to mark focal adhesions. Focal adhesion number and size were quantified using the NIH ImageJ software. Values were normalized to the vehicle ‘No Force’ condition. n >30 cells per condition from three independent experiments, * P <0.05 using Student’s t -test, scale bar=10 μm. Full size image PKA inhibits haemodynamic-induced focal adhesion growth Our data indicate that PKA is responsible for regulating matrix-dependent stiffening and focal adhesion growth in response to applied magnetic forces. However, the haemodynamic force of fluid shear stress is the critical physiological force in vivo . ECs subjected to shear stress remodel their focal adhesions in order to resist shear forces [21] , [22] , and PECAM-1 is part of a mechanosensory complex that influences cytoskeleton dynamics in ECs subjected to fluid shear stress [15] . Therefore, we extended our studies to investigate the role of the PKA pathway in EC focal adhesion dynamics in response to fluid shear stress. ECs plated on CL were subjected to shear stress (12 dyn cm −2 ) and immunostained for vinculin to highlight focal adhesions ( Fig. 6a ). ECs subjected to shear displayed a twofold increase in focal adhesion number ( Supplementary Fig. 5a ), consistent with previous reports [22] . Furthermore, we found that inhibition of PKA signalling significantly augmented shear-induced focal adhesion growth ( Fig. 4a ), similar to the growth of focal adhesions observed when tension was applied on PECAM-1 ( Fig. 5b ). It is important to note that inhibition of PKA did not significantly influence focal adhesion size or number in the absence of shear stress ( Supplementary Fig. 5b ). Next, we tested whether PECAM-1 was required for PKA-mediated suppression of focal adhesion growth by subjecting PECAM-1 −/− ECs to shear stress. Inhibition of PKA signalling did not affect focal adhesion growth in PECAM-1 −/− ECs (PECAM-1 knockout) in response to shear stress, whereas null cells engineered to re-express PECAM-1 displayed a significant increase in focal adhesion growth, similar to the effect seen in bovine aortic ECs ( Supplementary Fig. 6 , Fig. 6a ). Thus, these data indicate that PECAM-1-dependent PKA signalling regulates focal adhesion dynamics in response to the physiological stimulus of fluid shear stress. 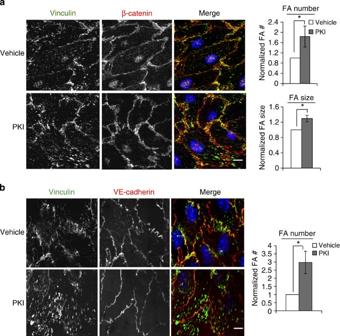Figure 6: The PKA pathway regulates haemodynamic-induced focal adhesion dynamicsin vitroandin vivo. (a) ECs adherent on CL pretreated with PKI (20 μM, 1 h) or vehicle and subjected to shear stress (12 dyn cm−2for 30 min). Cells were fixed and immunostained with anti-vinculin and anti-β-catenin antibodies. Focal adhesion number and size were quantified using the NIH ImageJ software. Values were normalized to the vehicle condition (n=3), *P<0.05 using a Student’st-test, scale bar=10 μm. (b) Vehicle or PKI (5 nmol) was administered to wild-type mice by retro-orbital injection. Two hours after injection, aortas were harvested anden facepreparations were immunostained with anti-vinculin and anti-VE-cadherin antibodies. Focal adhesions were quantified using the NIH ImageJ software. Values were normalized to the vehicle condition (n=4 mice/per group), *P<0.05 using a Student’st-test, scale bar=10 μm. Figure 6: The PKA pathway regulates haemodynamic-induced focal adhesion dynamics in vitro and in vivo . ( a ) ECs adherent on CL pretreated with PKI (20 μM, 1 h) or vehicle and subjected to shear stress (12 dyn cm −2 for 30 min). Cells were fixed and immunostained with anti-vinculin and anti-β-catenin antibodies. Focal adhesion number and size were quantified using the NIH ImageJ software. Values were normalized to the vehicle condition ( n =3), * P <0.05 using a Student’s t -test, scale bar=10 μm. ( b ) Vehicle or PKI (5 nmol) was administered to wild-type mice by retro-orbital injection. Two hours after injection, aortas were harvested and en face preparations were immunostained with anti-vinculin and anti-VE-cadherin antibodies. Focal adhesions were quantified using the NIH ImageJ software. Values were normalized to the vehicle condition ( n =4 mice/per group), * P <0.05 using a Student’s t -test, scale bar=10 μm. Full size image We sought to extend our in vitro shear stress studies to an in vivo setting. We examined focal adhesions in the descending aorta, as it is rich in CL composition and experiences relatively uniform shear stress patterns. In order to test whether PKA regulates focal adhesion growth in vivo , wild-type mice were injected with PKI or vehicle (dimethylsulphoxide). Two hours after injection, the descending aorta was harvested and en face preparations were immunostained for vinculin to highlight focal adhesions in the endothelium. Remarkably, inhibition of PKA signalling in vivo resulted in a significant increase in the number of focal adhesions present in the descending aorta ( Fig. 6b ) compared with control, suggesting that the PKA pathway is also a critical regulator of focal adhesion dynamics in ECs in the haemodynamic environment of the vessel. PKA promotes EC compliance in CL-rich regions of the aorta Several studies have suggested a link between vessel stiffness and cardiovascular disease [9] , [10] , [11] . However, measurements of EC stiffness ex vivo are lacking and the mechanisms that govern aortic EC stiffness remain largely unexplored. Our in vitro data suggest that growth of focal adhesions corresponds with a stiffer EC phenotype and that activation of the PKA pathway exerts a negative effect on active stiffening responses via inhibition of RhoA signalling. In contrast, suppression of PKA signalling restores mechanotransduction in response to tension on PECAM-1 ( Fig. 5 ), shear stress application in vitro ( Fig. 6a ) and in the haemodynamic environment of the blood vessel ( Fig. 6b ). In order to test the direct physiological relevance of these effects, we used external passive microbead rheology [23] to determine whether the PKA pathway is also a determinant of EC stiffness in vivo . The descending aorta was freshly isolated from control or PKI-treated mice 2 h after injection and prepared en face to expose the endothelium for passive microbead rheology measurements. The descending aorta was incubated with FN-conjugated beads in order to establish integrin-mediated attachments with the cortical actin cytoskeleton. Thermal motion of attached beads was tracked and the resulting mean-squared displacements (MSDs) were calculated for control or PKI-treated aortas ( Fig. 7a,b ). Of note, MSD trajectories show a slope less than unity (illustrated by black guideline in Fig. 7e ), indicating a subdiffusive viscoelastic response consistent with the movements of beads anchored to the actin cytoskeleton via integrins [24] . Ensemble-averaging of the bead populations revealed a significant decrease in MSD magnitude in PKI-treated descending aortas compared with control descending aortas ( Fig. 7e ). Furthermore, calculation of the average root mean squared (RMS) at the 1-s timescalefor each condition revealed a significant decrease in the effective radius of bead displacement in PKI-treated aortas ( Fig. 7f ). These data suggest a significant increase in stiffness in the endothelium of PKI-treated descending aortas compared with controls. Thus, the PKA pathway appears to be a significant regulator of EC stiffness in the CL-rich descending aorta. 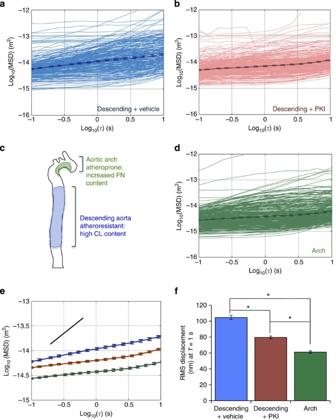Figure 7: The PKA pathway promotes EC compliance in atheroresistant regions of the aorta. (a) MSD trajectories of FN-conjugated, 4.5-μm beads attached to the atheroresistant region of the aorta. MSDs of individual curves (n>350 per condition, aggregated from three mice) are shown in light colour and the ensemble-average is represented by the dark curve with s.e.m. shown for indicated timescales. (b) MSD trajectories of FN-conjugated, 4.5-μm beads attached to the descending aorta from PKI-treated mice. MSDs of individual curves (n>350 per condition, aggregated from three mice) are shown in light colour and the ensemble-average is represented by the dark curve with s.e.m. shown for indicated timescales. (c) Diagram depicting ECM heterogeneity in the aorta. Regions of the aorta with high FN content are more prone to inflammation and disease, whereas regions with relatively high CL content are resistant to disease. (d) MSD trajectories of FN-conjugated, 4.5-μm beads attached to the atheroprone (aortic arch) regions of the aorta. MSDs of individual curves (n>350 per condition, aggregated from three mice) are shown in light colour and the ensemble-average is represented by the dark curve with s.e.m. shown for indicated timescales. (e) Ensemble-averaged MSDs of beads attached to endothelium of aortic preparations. Curves show a slope less than unity (illustrated by black guide line), indicating a subdiffusive viscoelastic response of beads anchored to the cortical actin cytoskeleton through apical integrin receptors. (f) RMS displacement at the 1-s timescale (τ=1 s) of beads attached to the endothelium in the descending aorta (+ vehicle or PKI) and the aorta arch, *P<0.0001 using a Student’st-test. Figure 7: The PKA pathway promotes EC compliance in atheroresistant regions of the aorta. ( a ) MSD trajectories of FN-conjugated, 4.5-μm beads attached to the atheroresistant region of the aorta. MSDs of individual curves ( n >350 per condition, aggregated from three mice) are shown in light colour and the ensemble-average is represented by the dark curve with s.e.m. shown for indicated timescales. ( b ) MSD trajectories of FN-conjugated, 4.5-μm beads attached to the descending aorta from PKI-treated mice. MSDs of individual curves ( n >350 per condition, aggregated from three mice) are shown in light colour and the ensemble-average is represented by the dark curve with s.e.m. shown for indicated timescales. ( c ) Diagram depicting ECM heterogeneity in the aorta. Regions of the aorta with high FN content are more prone to inflammation and disease, whereas regions with relatively high CL content are resistant to disease. ( d ) MSD trajectories of FN-conjugated, 4.5-μm beads attached to the atheroprone (aortic arch) regions of the aorta. MSDs of individual curves ( n >350 per condition, aggregated from three mice) are shown in light colour and the ensemble-average is represented by the dark curve with s.e.m. shown for indicated timescales. ( e ) Ensemble-averaged MSDs of beads attached to endothelium of aortic preparations. Curves show a slope less than unity (illustrated by black guide line), indicating a subdiffusive viscoelastic response of beads anchored to the cortical actin cytoskeleton through apical integrin receptors. ( f ) RMS displacement at the 1-s timescale ( τ =1 s) of beads attached to the endothelium in the descending aorta (+ vehicle or PKI) and the aorta arch, * P <0.0001 using a Student’s t -test. Full size image The aorta is heterogeneous in matrix composition, such that healthy, atheroresistant regions of the aorta (such as the descending aorta) are rich in CL content, whereas atheroprone regions of the aorta (such as the aortic arch) that are susceptible to inflammation and disease have a relatively high FN content ( Fig. 7c ). Our in vitro data suggest that, when tension is applied to PECAM-1, FN content promotes a stiffer EC phenotype, while stiffening is actively inhibited in ECs attached to CL. Therefore, we hypothesized that ECs located in atheroprone regions of the aorta would exhibit increased stiffness compared with ECs situated in atheroresistant regions. Atheroprone aortic arches were harvested, and external passive microbead rheology revealed a significant decrease in MSD magnitude in atheroprone regions of the aorta compared with atheroresistant regions ( Fig. 7d,e ). Furthermore, calculation of the RMS at the 1-s timescale revealed a significant decrease in the effective radius of bead displacement in atheroprone aortic arch compared with the atheroresistant descending aorta ( Fig.7f ). These data suggest a significant increase in stiffness in the ECs located in the FN-rich aortic arch, compared with ECs that reside within the CL-rich descending aorta. Given that inflammation and formation of atherosclerotic plaques preferentially develop in atheroprone regions of the vessel, such as the aortic arch, our data are also consistent with the idea that EC stiffness may be correlated to vascular disease. It is also important to note that inhibition of PKA signalling in the descending aorta increased EC stiffness values towards those observed in atheroprone regions of the aortic arch ( Fig. 7e,f ). Thus, our data indicate that PKA actively suppresses EC stiffening in healthy regions of the vessel and may play a critical role in maintaining vessel integrity in vivo . Here we identify a novel pathway that regulates endothelial mechanical responses and determines aortic EC stiffness, which may contribute to maintenance of blood vessel integrity. We sought out to determine the role of ECM identity in PECAM-1-mediated mechanotransduction and discovered that, while some responses are common, ECs adherent on CL display divergent signalling in response to mechanical tension on PECAM-1 compared with ECs adherent on FN. Although tension on PECAM-1 induces PI3K and downstream integrin activation, ECs on CL do not generate a stiffening response, which may be partially attributed to reduced focal adhesion remodelling. Mechanistically, we demonstrate that mechanical tension on PECAM-1 results in Gαs-mediated cAMP production, PKA activation and Ser188 phosphorylation of RhoA, which results in its deactivation. Inhibition of PKA signalling prolongs force-induced RhoA activation and results in cellular stiffening and focal adhesion growth in response to force ( Fig. 8 ). We further extended these findings to the physiological haemodynamic stimulus of fluid shear stress and reveal that PKA negatively regulates focal adhesion dynamics in ECs in vitro and in the haemodynamic environment of the vessel in vivo . Our in vivo studies suggest that this is a physiologically relevant signalling cascade, as ECs located in regions of the aorta where CL is the dominant ECM protein are more compliant than ECs located in FN-rich regions of the vessel. Finally, we highlight PKA as a critical regulator of EC mechanics in CL-rich regions of the aorta and demonstrate active regulation of aortic EC stiffness in vivo . 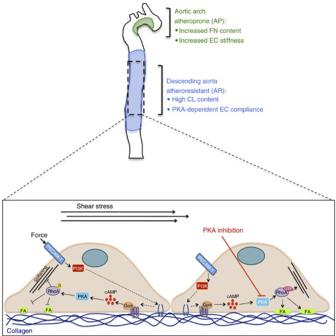Figure 8: Model of CL-dependent PECAM-1 mechanosignalling. PECAM-1-dependent mechanosignalling through CL-binding integrins results in Gαs-dependent PKA activation. PKA phosphorylates RhoA and inhibits its activity, which blunts EC stiffening responses. Inhibition of force-induced PKA activation promotes RhoA activation and is sufficient to restore the cellular response to force, including growth of focal adhesion and increased cellular stiffness. Figure 8: Model of CL-dependent PECAM-1 mechanosignalling. PECAM-1-dependent mechanosignalling through CL-binding integrins results in Gα s -dependent PKA activation. PKA phosphorylates RhoA and inhibits its activity, which blunts EC stiffening responses. Inhibition of force-induced PKA activation promotes RhoA activation and is sufficient to restore the cellular response to force, including growth of focal adhesion and increased cellular stiffness. Full size image PKA is a multifunctional protein that has many roles in cell biology. Within the endothelium, the kinase has well-documented roles in anti-inflammatory signalling [15] , angiogenesis [25] , barrier function [26] , [27] and cell migration [28] . Importantly, PKA-mediated RhoA inactivation has been shown to regulate endothelial barrier function in vitro [26] , and the kinase has been shown to tightly regulate RhoA activity during protrusion-retraction cycles in migrating cells [28] , [29] . In this study, we systemically delivered a PKI in order to examine effects on focal adhesion dynamics and EC compliance. Previous studies have demonstrated that inhibition of PKA signalling can promote inflammation and influence EC permeability [18] , [26] . It is possible that we could have affected these factors in our study, especially since EC stiffness and permeability are linked. However, our in vitro and in vivo studies clearly implicate PKA as a regulator of EC compliance. Future studies exploring the relationship between inflammation, EC compliance and permeability may provide valuable insights into factors that influence vessel health. Our in vitro studies also indicate that PKA inhibition of RhoA signalling influences EC responsiveness to force and focal adhesion dynamics. PKA can directly phosphorylate RhoA at serine 188, and phosphorylation of this residue inhibits activity of the GTPase [20] , [29] . Serine phosphorylation of RhoA increases its association with Rho-guanine dissociation inhibitor and negatively influences activity by sequestering the GTPase in the cytoplasm [30] . In addition to its role in regulating RhoA activity, a complex relationship between PKA and integrin-mediated adhesion also exists. Detachment of cells from the ECM triggers robust, but transient, activation of the kinase [31] , [32] . Conversely, integrin-mediated adhesion also stimulates PKA activation and is important for strengthening cell–cell and cell–matrix adhesions in certain cell types [33] . Our work highlights RhoA as a critical regulator of the cellular response to force. While mechanical stimulation of PECAM-1 induces RhoA activation in ECs adherent on CL, activation is transient and insufficient to initiate adaptive stiffening and focal adhesion growth. While we provide evidence for RhoA inactivation via serine phosphorylation, it is possible that force-dependent changes in GEF and GAP activity may also contribute to transient activation of the GTPase. For instance, p190RhoGAP is rapidly phosphorylated in ECs exposed to shear stress, and the GAP is required for flow-mediated changes in the actin cytoskeleton [34] . Therefore, it is possible that force-dependent activation of p190RhoGAP may also influence RhoA activity. In addition, previous work from our laboratory identified activation of the RhoGEF GEF-H1 in response to tension on PECAM-1 (ref. 12 ). Others have shown that PKA-dependent phosphorylation of GEF-H1 suppresses its GEF activity [35] . Therefore, it is also possible that force-dependent PKA activation inhibits GEF-H1-mediated GTP-loading at later time points. Nevertheless, our results clearly indicate that PKA regulates RhoA activity and the cellular response to mechanical force. Increased vessel stiffness is often associated with various vascular pathologies; therefore, understanding factors that contribute to EC stiffness in vivo is critical. Despite the association of vascular stiffness with disease, measurements of EC stiffness in vivo are lacking and mechanisms that regulate EC stiffness remain largely unexplored. Here we report that EC stiffness in vivo is heterogeneous and site-specific, such that ECs in FN-rich regions of the aorta prone to atherosclerosis are stiffer than those in atheroresistant regions. Furthermore, we identify PKA as an active regulator of EC compliance in atheroresistant regions of the aorta, as PKA inhibition promotes focal adhesion growth and increases EC stiffness in the descending aorta. The descending aorta is rich in CL composition and, notably, more resistant to atherosclerotic plaque development compared with other regions of the vasculature. In addition, vessel stiffness positively correlates with EC permeability and leukocyte transmigration [11] and, thus, contributes to the development of vascular disease. Therefore, PKA-mediated suppression of RhoA activity, inhibition of focal adhesion growth and increased EC compliance in the descending aorta may serve as a protective mechanism that maintains endothelial barrier function and regulates permeability. Overall, our work identifies a unique mechanosensitive and ECM-dependent signalling pathway that regulates EC stiffness and focal adhesion dynamics. Using magnetic tweezers, we show that tension on PECAM-1 initiates an intracellular signalling cascade that regulates the cellular force response and focal adhesion growth. We report that EC stiffness differs in regions of the aorta where different ECM compositions have been reported, and demonstrate that ECs in regions of the vessel that contain a high FN content are stiffer than those in CL-rich regions of the aorta. Furthermore, we identify PECAM-1-dependent PKA signalling as a critical regulator of focal adhesion dynamics and EC stiffness in vitro and in vivo , which may function as an atheroprotective mechanism in distinct regions of the vasculature. Cell culture and shear stress Bovine aortic ECs (a kind gift from Dr Shu Chien’s laboratory at UCSD) were maintained in Dulbecco’s modified Eagle’s medium (DMEM, Cellgro) with 10% fetal bovine serum (FBS) and 1% penicillin/streptomycin solution. PECAM-1 knockout and reconstituted cells were cultured in DMEM containing 10% FBS, 10 μM 2-mercaptoethanol (Invitrogen), 1 × nonessential amino acids (Invitrogen) and penicillin/streptomycin. Cells were plated on FN (10 μg ml −1 ) or Type I CL (40 μg ml −1 ) 4 h before experiments. For shear stress experiments, ECs were plated on 40 μg ml −1 CL in 0.5% FBS. Four hours after plating, cell slides were loaded on a parallel plate flow chamber in 0.5% FBS and 12 dynes cm −2 of shear stress was applied for indicated times, as previously described [36] . A surface area of 14 cm 2 on the BAEC-seeded slide was exposed to fluid shear stress generated by perfusing culture medium over the cells. The pH of the system was kept constant by gassing with 5% CO 2 /95% air and the temperature was maintained at 37 °C. Inhibitors and antibodies PKI was purchased from Calbiochem and was used at 20 μM for 1 h to inhibit PKA activity. The PECAM-1 antibody used for bead-coating (PECAM-1.3, 5 μg per 25 μl beads) was a generous gift from D.K. Newman (BloodCenter of Wisconsin). The RhoA antibody (26C4) used for western blotting (1:300) was purchased from Santa Cruz Biotechnology. The phospho-CREB (Ser133), phospho-PKA (Tyr197) and total PKA antibodies were from Cell Signaling and were used at 1:1,000 dilution for western blotting, and the phosphoserine antibody (1:1,000 dilution for western blot) and rhodamine–phalloidin (1:100 dilution for immunofluorescence) were from Invitrogen. The actin (1:2,000 dilution for immunoblot), vinculin (1:100 for immunofluorescence) and β-catenin (1:100 for immunofluorescence) antibodies and GDP-β-S (20 μM, 30 min) were obtained from Sigma, and the HUTS-4 antibody (which recognizes ligated β1 integrin) was purchased from Millipore and used at 1:100 dilution for immunofluorescence. The VE-cadherin antibody was from BD Pharmingen and was used at 1:100 dilution. RNA interference and transfections For RNA interference experiments, control (Dharmacon, siGLO RISC-free control siRNA), Gα s or PKA Cα siRNAs (Dharmacon) were transfected into cells using a calcium phosphate method. Briefly, 2.5 M CaCl 2 was added to siRNA (5 μM) diluted in 2 × HBS. The transfection mixture was mixed vigorously, incubated for 20 min at room temperature and added dropwise to plate containing 50% confluent cells. Cells were plated on CL 96 h post transfection and experiments were performed. The following siRNA sequences were used in this study: Gα s : 5′-CCACCAAAGUGCAGGACAUUU-3′; PKA Cα: 5′-GAGUAAAGGCUACAACAAAUU-3′. For GFP-PH experiments, cells were seeded at 50% confluence and transfected with 2.5 μg of the GFP-PH construct using Effectene reagents (QIAGEN) according to the manufacturer’s protocol. Experiments were performed 48 h after transfection. Preparation of beads Tosyl-activated paramagnetic beads (2.8 or 4.5 μm, Invitrogen) were washed with phosphate-buffered saline (PBS) and coated with an anti-PECAM-1 antibody (PECAM-1.3) or purified human FN according to the manufacturer’s protocol. Beads were quenched in 0.2 M Tris before use to remove any remaining tosyl groups and were resuspended in PBS or DMEM containing 10% FBS and 1% penicillin/streptomycin solution. Immediately before experiments, ECs were incubated with beads (two to six beads per cell) for 30 min at 37 °C. Cells were briefly washed with fresh media to remove unbound beads before force application. Pulsatile force application The UNC 3D Force Microscope was used to apply controlled pulsatile forces (~100 pN) to anti-PECAM-1-coated magnetic beads (2.8 μm diameter). Bead displacements were recorded with a high-speed video camera (Pulnix, JAI) and tracked using Video Spot Tracker (Computer Integrated Systems for Microscopy and Manipulation, http://cismm.cs.unc.edu/ ). Permanent force application For all immunostaining and biochemical analyses, continuous force (~10 pN) was applied to anti-PECAM-1-coated beads (4.5 μm diameter) using a permanent ceramic magnet (K&J Magnetics) parallel to the cell culture dish at a distance of 1 cm from the adherent cells. Immunofluorescence ECs grown on CL-coated cover slips and subjected to force (permanent magnet, 4.5 μm beads) were fixed for 20 min in PBS containing 2% formaldehyde, permeabilized with 0.2% Triton X-100 and blocked with PBS containing 10% goat serum for 1 h at room temperature. Antibody incubations were performed as previously described [12] . Briefly, cells were incubated with specific primary antibodies (1:100) overnight at 4 °C, briefly washed with PBS containing 0.001% Triton X-100 and then were incubated with a fluorescent secondary antibody for 1 h at room temperature. All cover slips were mounted in Vectashield mounting medium. Images were acquired using a confocal microscope (Olympus FV500) with a × 63 oil lens. cAMP measurements To assay cAMP, cells were lysed in 0.1 N HCl supplemented with 0.1% Triton X-100 for 10 min. Levels of cAMP were determined by competitive immunoassay (Sigma no. CA200) according to the manufacturer’s instructions. Samples were acetylated in order to increase assay sensitivity, and values were normalized to total protein levels. Rho pulldowns Adherent cells grown on ECM-coated 10-cm dishes were incubated with anti-PECAM-1-coated beads (4.5 μm, Invitrogen) for 30 min and subjected to force for indicated times. Briefly, following force application, cells were lysed in 50 mM Tris (pH 7.6), 500 mM NaCl, 1% Triton X-100, 0.1% SDS, 0.5% deoxycholate, 10 mM MgCl 2 and protease inhibitors. Anti-PECAM-1-coated magnetic beads were removed from lysates with a magnetic separator. Lysates were centrifuged for 5 min and supernatants were transferred to a new tube and incubated at 4° with 80 μg of purified (GST-RBD) bound to glutathione-sepharose beads. Bead pellets were washed in 50 mM Tris (pH 7.6), 150 mM NaCl, 1% Triton X-100, 10 mM MgCl 2 and protease inhibitors, and subsequently resuspended in Laemmli sample buffer and subjected to SDS–PAGE. Immunoprecipitation and western blotting Cells grown in 10-cm dishes and subjected to force as described above were harvested in lysis buffer (20 mM Tris (pH 7.4), 150 mM NaCl, 50 mM NaF, 1% NP-40) supplemented with 10 μg ml −1 aprotinin, 10 μg ml −1 leupeptin, 1 mM PMSF, 1 mM Na 3 VO 4 , 1 mM sodium pyrophosphate and 1 mM β-glycerophosphate. Lysates were pre-cleared with 15 μl protein A/G plus sepharose beads (Santa Cruz Biotechnology) for 1 h at 4 °C. Supernatants were then incubated with 30 μl protein A/G plus sepharose previously coupled to the primary antibodies for 3 h at 4 °C with continuous agitation. The beads were washed three times with lysis buffer supplemented with protease and phosphatase inhibitors and the immune complexes were eluted in 2 × SDS sample buffer. Associated proteins were subjected to SDS–PAGE and western blotting using the appropriate primary antibodies and IRDye-conjugated anti-mouse or anti-rabbit antibodies (Rockland). Images of western blotting were obtained with an Odyssey infrared scanner system. Quantification of integrin activation and focal adhesions ECs stained for ligated β1 integrin ( Supplementary Fig. 2B ) or vinculin were analysed with the NIH ImageJ software. Confocal image planes at the basal surface of the cell were chosen for analysis and RGB images were converted to 8-bit black and white images. Activated integrins and focal adhesions were defined by setting an intensity threshold to remove background signal. Integrin activation and focal adhesion size and number were analysed using the ‘Analyze particles’ function. Animals and en face aorta preparations All mice were used in accordance with the guidelines of the National Institutes of Health and the care and use of laboratory animals (approved by the Institutional Animal Care and Use Committees of the University of North Carolina at Chapel Hill). 5 nmol of PKI or dimethylsulphoxide was administered by retro-orbital injection into 10- to 14-week-old male C57BL/6 mice. Two hours after injection, descending aortas were isolated and processed for en face immunostaining. Briefly, the aorta was perfusion-fixed and dissected out under dissection microscope. The descending aortas were cut longitudinally and pinned flat with endothelium facing up on a Surperfrost/Plus glass slide (Fisher Scientific). Tissue sections were stained with anti-vinculin and anti-VE-cadherin antibodies and imaged as described above. Passive microbead assay for analysis of aortic ECs The aorta was freshly isolated and prepared en face on a cover slip. Briefly, the heart was perfused with PBS containing heparin and sodium nitroprusside and the live aorta was dissected out under a dissection microscope, cut longitudinally and mounted on a glass coverslip with the endothelium facing up. To anchor the aorta to the cover slip for experiments, a thin sheet (~20 × 40 × 2 mm) of polydimethylsiloxane rubber (Sylgard 184, Dow Corning) was positioned over the tissue. A small section (3 × 5 mm) of the polydimethylsiloxane sheet was removed before anchorage to serve as a media reservoir region of interest. The reservoir was immediately filled with Medium 199 containing 10% FBS and 15 mM HEPES in order to keep the tissue alive. FN-conjugated paramagnetic beads (4.5 μm, Invitrogen) were incubated over the endothelium for 20 min at 37 °C. The thermal motion of attached beads was imaged at × 40 using an upright reflective microscope (Orthoplan, Leitz) and recorded at 30 frames per second with a high-speed video camera (Pulnix, JAI). Bead motion was monitored for 1 min and tracked using Video Spot Tracker software (Computer Integrated Systems for Microscopy and Manipulation, http://cismm.cs.unc.edu/ ). The time-dependent MSD of the bead trajectories was computed using < r 2 (τ)>=<MSD>=<[ x ( t +τ)− x ( t )] 2 +[ y ( t +τ)− y ( t )] 2 >, where t is the elapsed time and τ is the time lag, or timescale. Beads included in analysis were separated from other beads by three bead diameters. Conditions were compared using the ensemble-averaged MSD and the RMS displacement. Statistical analysis Data are presented as means±s.e.m. P values were determined using a two-tailed unpaired Student’s t -test. How to cite this article: Collins, C. et al . Haemodynamic and extracellular matrix cues regulate the mechanical phenotype and stiffness of aortic endothelial cells. Nat. Commun. 5:3984 doi: 10.1038/ncomms4984 (2014).